Multiple S-isotopic evidence for episodic shoaling of anoxic water during Late Permian mass extinction Global fossil data show that profound biodiversity loss preceded the final catastrophe that killed nearly 90% marine species on a global scale at the end of the Permian. Many hypotheses have been proposed to explain this extinction and yet still remain greatly debated. Here, we report analyses of all four sulphur isotopes ( 32 S, 33 S, 34 S and 36 S) for pyrites in sedimentary rocks from the Meishan section in South China. We observe a sulphur isotope signal (negative δ 34 S with negative Δ 33 S) that may have resulted from limitation of sulphate supply, which may be linked to a near shutdown of bioturbation during shoaling of anoxic water. These results indicate that episodic shoaling of anoxic water may have contributed to the profound biodiversity crisis before the final catastrophe. Our data suggest a prolonged deterioration of oceanic environments during the Late Permian mass extinction. The end-Permian extinction has been regarded as the most severe of all mass extinctions in the Phanerozoic [1] , [2] , [3] . Exterrestrial impact, the eruption of Siberian basalts, oceanic anoxia, hydrogen sulphide poisoning or perhaps combination of these has been proposed to explain this extinction [1] , [2] , [3] , [4] , [5] , [6] , [7] . However, the cause of biodiversity crisis before the final catastrophe has received little attention. To explore palaeoceanographic changes and their contributions to the Late Permian mass extinction, we analysed all four S-isotopic compositions of pyrites from the Meishan section in South China. The Meishan section arguably provides the most detailed records of the Latest Permian biotic crisis [1] , [8] , [9] . A profound loss of marine fauna, including most fusulinids and ammonoids and many brachipods, is observed below Bed 25 at Meishan [8] , [9] , [10] . Fossil records suggest that the onset of biodiversity loss probably began during deposition of Bed 22, with an extinction rate of <33% (ref. 8 , 9 , 10 ; Em in Fig. 1 ), and continued until the end-Permian extinction event, which is preserved in Beds 25–26 (E1 in Fig. 1 ). At Meishan, the end-Permian extinction preserved by Beds 25–26 is estimated to have marked a loss of 94% of marine species within <0.5 million years [8] , [11] . Recent biomarker data also suggest a separate, later episode of extinction occurring during deposition of Bed 28 (ref. 12 ; E2 in Fig. 1 ). The picture that has emerged may not be of a singular event but rather of a series of events, the cause(s) of which is currently the most debated of the mass extinctions. 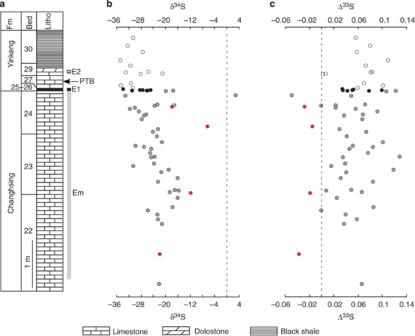Figure 1: The Permian–Triassic stratigraphy and sulphur isotopic data at Meishan. (a) Stratigraphy of the Permian–Triassic boundary (PTB) and extinction events Em, E1 and E2. Note that E2 corresponds to Bed 28 (not shown). (b) Sulphur isotopic compositions (δ34S) of pyrites at Meishan. Grey filled circles are Beds 22–24, black circles are Beds 25–26 and open circles are Beds 27–30. (c) Sulphur isotopic compositions (Δ33S) of pyrites at Meishan. Red circles indicate negative δ34S and Δ33S values. Figure 1: The Permian–Triassic stratigraphy and sulphur isotopic data at Meishan. ( a ) Stratigraphy of the Permian–Triassic boundary (PTB) and extinction events Em, E1 and E2. Note that E2 corresponds to Bed 28 (not shown). ( b ) Sulphur isotopic compositions (δ 34 S) of pyrites at Meishan. Grey filled circles are Beds 22–24, black circles are Beds 25–26 and open circles are Beds 27–30. ( c ) Sulphur isotopic compositions (Δ 33 S) of pyrites at Meishan. Red circles indicate negative δ 34 S and Δ 33 S values. Full size image Among all extinction events at Meishan (Em–E2), the end-Permian extinction at Beds 25–26 has been examined in greatest detail. The catastrophic extinction event (E1 in Fig. 1 ) coincides with many geochemical anomalies, such as a negative δ 13 C excursion [8] , [12] , [13] , the presence of a relatively large fractionation of 45.3‰ between pyrite and carbonate-associated sulphate [14] , the possible existence of fullerenes in the boundary sediments [15] (but see refs. 16 , 17 ), negative δ 34 S shift for carbonate-associated sulphate [18] (but see ref. 19 ) and the occurrence of isorenieratane [20] , [21] , [22] , [23] (but see ref. 24 ). Hypotheses about the cause of extinction have been proposed on the basis of these records and include impact, chemocline upward excursion, photic zone euxinia (anoxic and sulphidic water column conditions) or some combinations of these [1] . It remains unclear which of these hypotheses are valid and the nature of their connection to the profound biodiversity loss that preceded the end-Permian extinction. In this study, we report multiple S-isotopic analysis of pyrites from the Meishan section. We discover a sulphur isotope signal (negative δ 34 S with negative Δ 33 S) that suggests episodes when porewater sulphate was converted nearly quantitatively to sulphide. This S-isotopic signal may have resulted from mixing of pyrites and suggests that shoaling of deep anoxic water may have contributed to the significant biodiversity loss before the final catastrophic extinction. Sampling of the Meishan section Our samples were collected from the Meishan section in South China, which is the Global Stratotype Section and Point (GSSP) for the Permian–Triassic boundary [8] , [9] . We sampled Beds 22–30 of the Late Permian Changhsing Formation to Early Triassic Yinkeng Formation that recorded the detailed patterns of the Late Permian extinction ( Fig. 1 ). Beds 22–24 comprises limestone. Beds 25 and 26 were named 'event beds', which were usually ∼ 1–2 cm thick, among which bed 25 was gray-green clay and bed 26 was black clay. Zircons from ash layers in Beds 25–26 yielded a U-Pb age of 251.4±0.3 Ma (ref. 11 ). Bed 27 consists of argillaceous wackstone and dolostone within which the first appearance datum of conodont Hindeodus parvus was reported ( ∼ 10 cm above Bed 25), marking the Permian–Triassic boundary [9] . Bed 28 is gray-green ash clay of ∼ 0.5 cm thickness from which a U-Pb age of 250.7±0.3 Ma of zircon was obtained [11] . The lower part of Bed 29 is dominated by carbonate and overlain by organic-rich mudstone up to Bed 30 ( Fig. 1 ). S-isotopic data before the end-Permian extinction We report data for all four S-isotopes ( 32 S, 33 S, 34 S and 36 S) of pyrites from the Meishan section, which is the first multiple S-isotopic study on the Permian–Triassic mass extinctions. Sulphur isotope data are presented using delta notation δ 34 S=[( 34 S/ 32 S) sample /( 34 S/ 32 S) reference −1] and capital delta notation Δ 33 S=[( 33 S/ 32 S) sample /( 33 S/ 32 S) reference −(( 34 S/ 32 S) sample /( 34 S/ 32 S) reference ) 0.515 ]. Capital delta and delta values are given in units of per mil (‰). Small deviations for Δ 33 S and Δ 36 S can be used to examine the way in which sulphur is cycled in biological and biogeochemical systems [25] , [26] , [27] , [28] , [29] . Figures 1 and 2 (full analytical data available as Supplementary Data 1 ) present the δ 34 S and Δ 33 S data for pyrites from the Meishan section. 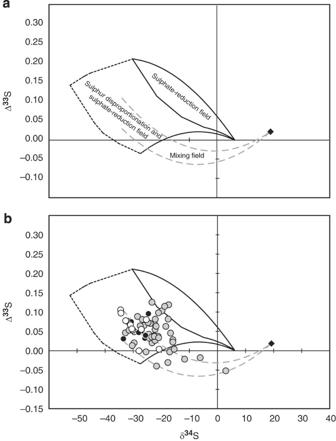Figure 2: Plot of Δ33S against δ34S. (a) Plot of Δ33S against δ34S illustrating fields of data produced by sulphate reduction only, sulphate reduction and disproportionation, and mixing between pyrite produced by near quantitative reduction of sulphate and by a combination of sulphate reduction and disproportionation. (b) Plot of Δ33S against δ34S for data from Meishan pyrites illustrating data that get plotted in fields of sulphate reduction and disproportionation, and also mixing between pyrite produced by near quantitative reduction of sulphate and by a combination of sulphate reduction and disproportionation. Grey filled circles are Beds 22–24, black circles are Beds 25–26 and open circles are Beds 27–30. Figure 2: Plot of Δ 33 S against δ 34 S. ( a ) Plot of Δ 33 S against δ 34 S illustrating fields of data produced by sulphate reduction only, sulphate reduction and disproportionation, and mixing between pyrite produced by near quantitative reduction of sulphate and by a combination of sulphate reduction and disproportionation. ( b ) Plot of Δ 33 S against δ 34 S for data from Meishan pyrites illustrating data that get plotted in fields of sulphate reduction and disproportionation, and also mixing between pyrite produced by near quantitative reduction of sulphate and by a combination of sulphate reduction and disproportionation. Grey filled circles are Beds 22–24, black circles are Beds 25–26 and open circles are Beds 27–30. Full size image The δ 34 S of pyrites in Beds 22–24 of the Changhsing Formation show significant negative values ranging from −6.26 to −33.0‰ (mostly −17 to −31‰) except one positive value of 2.88‰ in the uppermost part of Bed 24 ( Fig. 1 ). Δ 33 S values of pyrites from Bed 22 to Bed 24 range from 0.123 to −0.037. For most of the Changhsing pyrites, they show negative δ 34 S values and positive Δ 33 S values ( Fig. 2b , quadrant II). A positive δ 34 S value of 2.88‰ with negative Δ 33 S value of −0.049 for pyrite is seen in the uppermost part of Bed 24 ( Fig. 2b , quadrant IV). Negative δ 34 S values and negative Δ 33 S values are present for Beds 22–24 ( Fig. 2b , quadrant III) and they occur scattered through the Changhsing Formation ( Fig. 1 ). S-isotopic data during and after the end-Permian extinction The δ 34 S of pyrites in Beds 25–26, where the final catastrophic extinction occurred, exhibit negative values ranging from −33.72 to −24.78‰, with positive Δ 33 S values ranging from 0.034 to 0.010 ( Fig. 2b , quadrant II). Above the extinction event at Beds 25–26, pyrites from Bed 27 to Bed 30 of the Yinkeng Formation are characterized by significantly negative δ 34 S values from −21.0 to −34.7‰ and Δ 33 S values from 0 to 0.101 ( Fig. 2b , quadrant II). We observe no pyrites from Bed 25 to Bed 30 of the Yinkeng Formation showing negative δ 34 S and negative Δ 33 S. A context for interpreting these observations is presented in Figure 2 , in which we illustrate the predictions of a steady-state global sulphur cycle model similar to that described by Johnston et al . [30] . The fields in this figure represent the composition of the global average of buried pyrite and do not account for heterogeneity of sedimentary pyrite on basinal or regional scale. The fields of buried pyrite are situated in quadrant II (negative δ 34 S and positive Δ 33 S), and its location is a consequence of the fractionation relationships produced by sulphate reduction, disproportionation of sulphur intermediate compounds and the conservation of mass in the sulphur cycle [31] . This pyrite may be formed in water columns or in sediments (so-called syngenetic pyrite or diagenetic pyrite), and the negative δ 34 S and positive Δ 33 S values reflect lower degrees of sulphate reduction in open-system environments, and pyrite with this composition is typical in modern sediments and geological rock record [30] , [32] , [33] . Observation of pyrite that does not get plotted in this field reflects local and regional processes that operate in the sulphur cycle. For example, diagenetic pyrite formed in normal marine sediments with positive δ 34 S and either positive or negative Δ 33 S (quadrant I and IV) reflects high degrees of sulphate reduction or an approach to quantitative reduction of sulphate [29] , [32] . Pyrite with negative δ 34 S and negative Δ 33 S values in quadrant III cannot, however, be accounted for neither by sulphate reduction or sulphur disproportionation in typical stable diagenetic systems nor by nearly quantitative reduction of sulphate that acts alone. Pyrite with negative δ 34 S and negative Δ 33 S (quadrant III) suggests mixing of sulphur from sulphide sources with sulphur from nearly quantitative reduction of sulphate [29] , [32] . This latter isotopic signature is present in some pyrites from Meishan, which temporally correlate with profound biodiversity loss ( Fig. 2 ) and provide new insights into palaeoceanographic changes during the Late Permain extinction processes. The majority of pyrite analyses occupy quadrant II, showing significant negative δ 34 S values and positive Δ 33 S values observed from the Changshing and Yinkeng formations ( Fig. 2b ) and are consistent with observations from other diagenetic settings in both euxinic and oxic environments [33] . One analysis occupies quadrant IV ( ∼ 9 cm below Bed 25), showing a positive δ 34 S of 2.88‰ and negative Δ 33 S of −0.049 ( Fig. 2b ). This isotopic composition has more negative δ 34 S and Δ 33 S than estimates of contemporaneous seawater [34] , and it suggests mixing between an end-member with little or no isotopic fractionation during sulphate reduction or nearly quantitative reduction of sulphate. Such mixing can occur when sulphate-reduction rates are enhanced relative to the supply of porewater sulphate ( Fig. 2 ). We suggest that the four analyses with negative δ 34 S and negative Δ 33 S values located in quadrant III ( Fig. 2b ) reflect a similar situation. These isotopic characteristics are present episodically from Beds 22 to 24, and suggest mixing of pyrite produced in two different settings, one in which sulphate is nearly quantitatively reduced and the other in which sulphate reduction and pyrite formation occurs with significant exchange between porewater sulphate in sediment and sulphate in the overlying water column. The mixing of pyrite observed from Meishan may be indicative of shoaling of anoxic deep water before the end-Permian mass extinction in Beds 25–26. 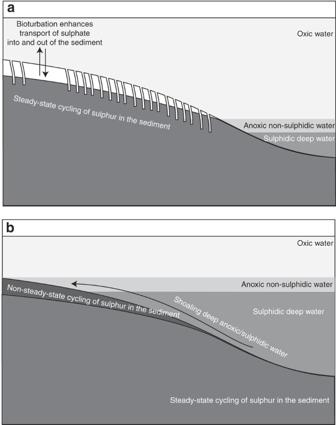Figure 3: A cartoon representing the sulphur cycle associated with the shoaling deep anoxic water during the Latest Permian. (a) Sulphur cycle under typical steady-state conditions in which bioturbation aerates shallow sediments and promotes transport of sulphate into and out of the sediments. (b) Sulphur cycle associated with shoaling of deep anoxic water in which bioturbation shuts down, limiting transport of sulphate within sediments and exchange between sediment pore water sulphate and oceanic sulphate pools. High organic content in the sediments promotes nearly quantitative sulphate reduction, resulting in non-steady-state conditions and formation of pyrites with negative δ34S and negative Δ33S values as seen inFigures 1and2. A cartoon that describes the principal features of this hypothesis is presented in Figure 3 , and envisions a situation similar to that observed in the Black Sea where oxic waters overly but is separated from a deep water euxinic pool by Fe 2+ -rich non-sulphidic, anoxic waters ( Fig. 3a ). This scenario is based on deep-water column euxinia during the latest Permian that has been well documented [2] , [5] , [14] , [35] , [36] . When anoxic water shoal, the sulphur cycle within sediments, formerly in the oxic zone, will change from a system with effective transport of sulphate into and out of the sediment ( Fig. 3b ) to a system in which bioturbation does not play a significant role, and effective exchange of sulphate between the sediment porewater and the overlying water column would be suppressed. Figure 3: A cartoon representing the sulphur cycle associated with the shoaling deep anoxic water during the Latest Permian. ( a ) Sulphur cycle under typical steady-state conditions in which bioturbation aerates shallow sediments and promotes transport of sulphate into and out of the sediments. ( b ) Sulphur cycle associated with shoaling of deep anoxic water in which bioturbation shuts down, limiting transport of sulphate within sediments and exchange between sediment pore water sulphate and oceanic sulphate pools. High organic content in the sediments promotes nearly quantitative sulphate reduction, resulting in non-steady-state conditions and formation of pyrites with negative δ 34 S and negative Δ 33 S values as seen in Figures 1 and 2 . Full size image When anoxic deep water shoal into the oxic zone, oxidation of sulphide in the sediment will be suppressed and there is a potential for delivery of iron to the sediment from the anoxic water column ( Fig. 3b ). The sediments in which sulphate reduction is initiated may possess significant organic electron donors for sulphate reduction, allowing for high sulphate-reduction rates that may outpace the sulphate supply by diffusion from the overlying water column, thus contributing a sulphur component that occupies quadrant III and IV. Shoaling of anoxic water would have killed marine animals, limiting bioturbation, transport of sulphate from overlying seawater into the sediments and sulphide oxidation. Addition of pyrite formed during such an event to pyrite already present in the sediments would therefore provide an explanation for our observations of pyrite that get plotted in quadrant IV and pyrite that get plotted in quadrant III (Beds 22–24; Fig. 2 ). The negative δ 34 S and negative Δ 33 S values at Beds 22–24 from Meishan therefore provide a geochemical signal that links episodic incursion of anoxic water with extermination of bioturbating organisms, suppression of sulphate transport and enhanced sulphate reduction. The temporal coincidence between shoaling of anoxic water and the profound biodiversity loss suggests that episodic incursion of anoxic water into the shallower water may have contributed to the biodiversity crisis that preceded the end-Permian extinction. Interestingly, we observe no negative δ 34 S and negative Δ 33 S values at Beds 25–26 that recorded the final catastrophic extinction. This may be attributable to preservation biases at Meishan but it may also reflect a stable diagenetic system and imply that the cause of the end-Permian extinction was different from that of the biodiversity loss before it. Further isotopic studies carried out in the framework of biostratigraphy should clarify the relationships between environmental changes and the Late Permian mass extinction. Pyrite extraction In this study, pyrite sulphur from rock samples was extracted using chromium reduction and converted to silver sulphide. During this procedure, the product H 2 S was carried by nitrogen gas through a condenser and a bubbler filled with milli-Q water, and collected as zinc sulphide by reaction with a slightly acidic Zn-acetate solution. The zinc sulphide was made to react with silver nitrate to yield silver sulphide, which was collected by centrifugation and washed with successive rinses of milli-Q water, ammonium hydroxide solution and milli-Q water. Sulphur isotopic analysis Silver sulphide (Ag 2 S) was converted to SF 6 by a fluorination reaction with a fivefold excess of F 2 at 250 °C for 8 h in a Ni reaction vessel. After the reaction, product SF 6 was condensed from the residual F 2 into a liquid-nitrogen-cooled trap (−177 °C). The F 2 was removed to another part of the manifold where it was passivated by reaction with hot KBr. The SF 6 was subsequently thawed to room temperature and then cooled to −111 °C to condense contaminants, such as trace HF, before it was transferred to the injection loop of a gas chromatograph, which was cooled to −177 °C. Gas chromatograph purification of SF 6 was undertaken using a composite column consisting of a 1/8-inch diameter, 6-foot lead column of 5A molecular sieve, followed by a 1/8-inch diameter, 12-foot-long Haysep-Q™ column. The He carrier flow was set at 20 ml min −1 . The SF 6 peak was registered on a thermal conductivity detector and then isolated by freezing into a liquid-nitrogen-cooled trap. The isotopic composition of the purified SF 6 was determined by dual-inlet gas-source mass spectrometry monitoring ion beams at m / e of 127, 128, 129 and 131, using a Thermo Finnigan MAT 253 gas source mass spectrometer. One-sigma uncertainties on mass-dependent reference materials are better than ±0.2‰, ±0.01‰ and ±0.2‰ in δ 34 S, Δ 33 S and Δ 36 S, respectively. Uncertainties on the measurements reported here are estimated to be better than ±0.2‰, ±0.01‰ and ±0.2‰. The results of our measurements are presented in Supplementary Data 1 . How to cite this article: Shen, Y. et al . Multiple S-isotopic evidence for episodic shoaling of anoxic water during Late Permian mass extinction. Nat. Commun. 2:210 doi: 10.1038/ncomms1217 (2011).